The bacterial metabolite 2-aminoacetophenone promotes association of pathogenic bacteria with flies Bacteria contaminate insects and secrete metabolites that may affect insect behaviour and potentially fitness through unknown mechanisms. Here we show that the ‘grape-like’ odorant 2-aminoacetophenone (2AA), secreted by Pseudomonas aeruginosa (a ubiquitous opportunistic human pathogen), facilitates attraction to food for several fly species including Musca domestica, Ceratitis capitata and Drosophila melanogaster. Constant feeding on 2AA increases the level of long-term colonization of the flies’ intestine by P. aeruginosa . Odour perception is necessary for enhanced attraction to food containing 2AA, and expression in the Drosophila olfactory organs of odorant receptors Or49b and Or10a potentiates, while expression of Or85a inhibits, preference for 2AA. Our study shows that 2AA lures the flies to the bacterial source and increases the extent of colonization of the fly intestine by the bacteria that produce it, as a means to facilitate bacterial dissemination to new locations. Insects are notorious for transmitting infectious diseases. Diptera in particular are susceptible to colonization by various human pathogens. Houseflies ( Musca domestica ), for example, often feed on faecal waste and garbage and carry microbes, such as pathogenic Escherichia coli and Pseudomonas aeruginosa , on their outer surface and in their gut [1] , [2] , [3] . The Mediterranean fruit fly Ceratitis capitata might also carry and transmit pathogenic E. coli and P. aeruginosa ( P.a ) [4] , [5] , while the fruit fly Drosophila melanogaster might carry Pseudomonas species in nature, which colonize and induce pathology in flies [6] , [7] . P.a is an opportunistic pathogen and a common inhabitant of soil and water [8] . These bacteria are essentially ubiquitous, found regularly on plant surfaces and occasionally on animals [9] . Humans too are occasional carriers of P.a , and wound-infected and severely immunocompromised individuals are particularly susceptible to infection [9] , [10] . While bacteria contaminate flies by targeting fly habitats and fly food, attraction of flies by the bacteria themselves may aid colonization. For example, bacteria and their products have been shown to attract various Diptera species, including fruit flies, screw-worm flies, apple maggots and mosquitoes [11] , [12] , [13] , [14] , [15] . Yet in those studies, the mechanisms attracting flies remain obscure or those proposed apply only to specific insect families. Moreover, evidence suggests that microbially contaminated food repels insects from feeding on it, because they have developed behavioural defence mechanisms against infection [16] , [17] . Here we studied the ability of 2-aminoacetophenone (2AA), a secondary metabolite of P.a , to induce the association between bacteria and flies. 2AA is a single benzene ring aromatic compound with a ‘grape-like’ odour that promotes chronic P.a infection phenotypes, including long-term bacterial survival at a stationary phase and a reduction in bacterial virulence in various hosts [18] . We assess the ability of 2AA to attract flies and to facilitate intestinal colonization by P.a upon 2AA ingestion. We find that 2AA acts both as an odorant attractant and as a facilitator of intestinal colonization in several fly species, including M. domestica, C. capitata and D. melanogaster . D. melanogaster attraction to 2AA To assess if D. melanogaster can sense P.a in its food, we devised a dual small fly trap system ( Fig. 1a ) allowing flies to choose between a sterile agar medium and an agar medium containing fully-grown P.a . We found that more flies entered traps where P.a was grown ( Fig. 1b ). Similarly, flies preferred traps containing P.a liquid cultures added to live yeast paste versus traps containing only live yeast paste ( Fig. 1c ). It has previously been shown that D. melanogaster is attracted to grapes and wine, some varieties of which contain 2AA [19] . We examined if flies are also attracted to P.a because these bacteria are known to secrete the ‘grape-like’ odorant 2AA [20] . Using a P.a gene deletion strain that inhibits the production of 2AA, we find that D. melanogaster prefers yeast paste containing bacteria that produce 2AA over those that do not produce 2AA ( Fig. 1d ). To determine whether the mere presence of 2AA in the food enhances fly attraction to it, we added pure 2AA on yeast paste and found that twice as many flies preferred 2AA over the no-2AA control ( Fig. 1e ). Similarly, glass traps filled with diluted molasses and placed in an olive grove ( Fig. 1f ) collected on an average fewer individual D. melanogaster than equivalent traps supplemented with 2AA ( Fig. 1g ). Thus 2AA and the bacteria that produce it attract D. melanogaster to food. 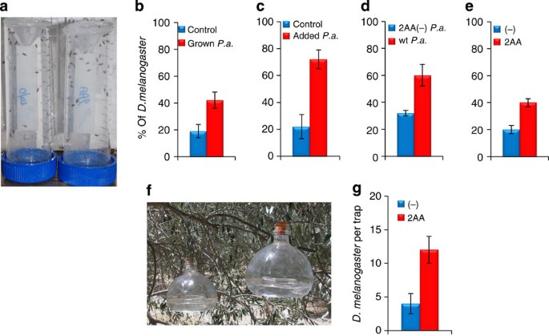Figure 1:D. melanogasterattraction to 2AA. (a) Dual small fly trap forD. melanogasterfood source attraction assessment. (b)D. melanogasterattraction to agar medium on whichP. aeruginosa(P.a.) grows. (c)D. melanogasterattraction to yeast paste on whichP. aeruginosaculture was added. (d)D. melanogasterattraction to yeast paste on which 2AA-producingP. aeruginosaculture was added versus culture that does not produce 2AA. (e)D. melanogasterattraction to yeast paste on which pure 2AA was added. (f) Example of liquid filled glass traps placed in an olive grove. (g) IncreasedD. melanogasternumbers in glass traps containing 2AA. Inb–e, 100 flies were used per each of then=6 replicates; ing,n=6 replicates; error bars represent s.d. Differences inb–e(usingt-test) and ing(usingχ2-test) are significant,P<0.01. Figure 1: D. melanogaster attraction to 2AA. ( a ) Dual small fly trap for D. melanogaster food source attraction assessment. ( b ) D. melanogaster attraction to agar medium on which P. aeruginosa ( P.a. ) grows. ( c ) D. melanogaster attraction to yeast paste on which P. aeruginosa culture was added. ( d ) D. melanogaster attraction to yeast paste on which 2AA-producing P. aeruginosa culture was added versus culture that does not produce 2AA. ( e ) D. melanogaster attraction to yeast paste on which pure 2AA was added. ( f ) Example of liquid filled glass traps placed in an olive grove. ( g ) Increased D. melanogaster numbers in glass traps containing 2AA. In b – e , 100 flies were used per each of the n =6 replicates; in g , n =6 replicates; error bars represent s.d. Differences in b – e (using t -test) and in g (using χ 2 -test) are significant, P <0.01. Full size image The attraction of M. domestica , C. capitata and Bactrocera oleae to 2AA Next we sought to assess if flies belonging to other Diptera families, specifically M. domestica and C. capitata , commonly reported as carriers of P.a [1] , [2] , [3] , [4] , [5] , are also attracted by bacteria that produce 2AA. We devised a dual big fly trap system ( Fig. 2a ) and found that M. domestica preferred live yeast paste that contained P.a over yeast paste containing no bacteria ( Fig. 2b ). M. domestica also preferred live yeast paste containing a P.a strain that produces 2AA over another that does not ( Fig. 2c ). Finally, M. domestica preferred live yeast paste containing pure 2AA over no-2AA yeast paste ( Fig. 2d ). Using a similar dual big fly trap system ( Fig. 2e ), we noticed that C. capitata preferred live yeast paste containing a P.a strain that produces 2AA over another that does not ( Fig. 2f ) and yeast paste containing pure 2AA over no-2AA yeast paste ( Fig. 2g ). To assess if flies prefer fruits on trees treated with 2AA, we used wild-caught olive-infesting B. oleae ( Fig. 2h ), a species belonging to the same family with C. capitata [21] . We found that olives of 10 young olive trees sprayed with 2AA were more intensively infested than olives of 10 control-water sprayed trees, bearing 759 versus 321 total stings, respectively ( χ 2 -test, P <0.001; Fig. 2i ). 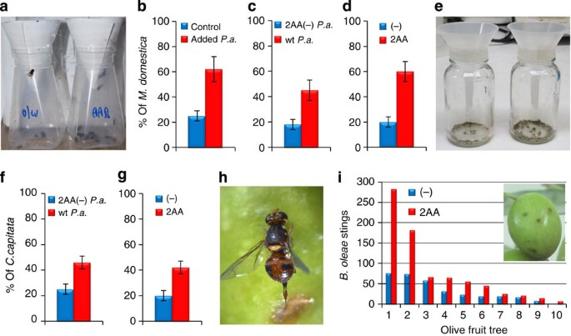Figure 2:M. domestica,C. capitataandB. oleaeattraction to 2AA. (a) Dual big fly trap forM. domesticafood source attraction assessment. (b)M. domesticaattraction to yeast paste on whichP. aeruginosa(P.a.) culture was added. (c)M. domesticaattraction to yeast paste on which 2AA-producingP. aeruginosaculture was added versus culture that does not produce 2AA. (d)M. domesticaattraction to yeast paste on which pure 2AA was added. (e) Dual big fly trap forC. capitatafood source attraction assessment. (f)C. capitataattraction to yeast paste on which 2AA-producingP. aeruginosaculture was added versus culture that does not produce 2AA. (g)C. capitataattraction to yeast paste on which pure 2AA was added. Inb–dandf,g, 50 and 100 flies respectively were used per each replicate (n=6); error bars represent s.d. (h) Wild-caughtB. oleaelanded on a stung olive fruit. (i) Total stings per each of the 10 trees sprayed with water (−) versus the 10 trees sprayed with water plus 2AA. Inset shows olive fruit bearing four stings. Differences shown inb–d,f,g(usingt-test) andi(usingχ2-test) are siginificant,P<0.01. Figure 2: M. domestica , C. capitata and B. oleae attraction to 2AA. ( a ) Dual big fly trap for M. domestica food source attraction assessment. ( b ) M. domestica attraction to yeast paste on which P. aeruginosa ( P.a. ) culture was added. ( c ) M. domestica attraction to yeast paste on which 2AA-producing P. aeruginosa culture was added versus culture that does not produce 2AA. ( d ) M. domestica attraction to yeast paste on which pure 2AA was added. ( e ) Dual big fly trap for C. capitata food source attraction assessment. ( f ) C. capitata attraction to yeast paste on which 2AA-producing P. aeruginosa culture was added versus culture that does not produce 2AA. ( g ) C. capitata attraction to yeast paste on which pure 2AA was added. In b – d and f , g , 50 and 100 flies respectively were used per each replicate ( n =6); error bars represent s.d. ( h ) Wild-caught B. oleae landed on a stung olive fruit. ( i ) Total stings per each of the 10 trees sprayed with water (−) versus the 10 trees sprayed with water plus 2AA. Inset shows olive fruit bearing four stings. Differences shown in b – d , f , g (using t -test) and i (using χ 2 -test) are siginificant, P <0.01. Full size image Colonization of infected flies in the presence of 2AA Subsequently, we sought to assess if exposure of flies to P.a -contaminated food resulted in fly contamination and concomitant bacterial dissemination to new locations. We compared D. melanogaster feeding on a sucrose medium mixed with bacterial cultures that contained bacterially produced 2AA with those that did not contain 2AA. We found that each exposed fly carried 100–1,000 P.a cells on its surface and ~10 5 in its gut irrespective of the presence of 2AA in the fly food ( Fig. 3a ). Moreover, each exposed fly transferred >1,000 P.a cells onto sterile paper discs within 24 h ( Fig. 3a ). Similarly, each P.a -exposed C. capitata fly carried 10–100 P.a cells on its surface, ~10 5 inside its gut and transferred 100–1,000 cells onto sterile paper discs irrespective of the presence of 2AA in the fly food ( Fig. 3b ). Thus flies reaching their food get sufficiently contaminated with bacteria, which they may then transmit to new areas within their environment. 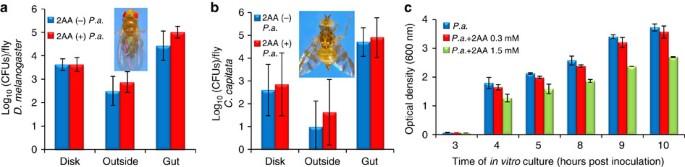Figure 3: Fly short-term colonization, bacteria dissemination andin vitrogrowth ofP. aeruginosain the presence of 2AA. (a,b) Bacterial load on the outside, the gut and on clean discs on whichD. melanogaster(a) orC. capitata(b) were transferred. Flies were initially fed on a 2AA-producingP. aeruginosaculture or a culture that does not produce 2AA. (c) Optical density of LB medium cultures inoculated with 107P. aeruginosacells per ml and left to grow in the presence of various concentrations of 2AA. Foraandb,n=9 fly samples (three flies per sample) andn=6 discs, and forc,n=7 replicate cultures were assessed; error bars represent s.d. Figure 3: Fly short-term colonization, bacteria dissemination and in vitro growth of P. aeruginosa in the presence of 2AA. ( a , b ) Bacterial load on the outside, the gut and on clean discs on which D. melanogaster ( a ) or C. capitata ( b ) were transferred. Flies were initially fed on a 2AA-producing P. aeruginosa culture or a culture that does not produce 2AA. ( c ) Optical density of LB medium cultures inoculated with 10 7 P. aeruginosa cells per ml and left to grow in the presence of various concentrations of 2AA. For a and b , n =9 fly samples (three flies per sample) and n =6 discs, and for c , n =7 replicate cultures were assessed; error bars represent s.d. Full size image Because 2AA could affect bacterial growth directly, we assessed the in vitro growth of bacteria in the presence of 2AA. We found that P.a growth was equal or slower in cultures in which 2AA was added into the bacterial medium ( Fig. 3c ), suggesting that 2AA does not promote bacterial growth directly. In addition, we assessed whether 2AA consumption affects bacterial persistence in the fly gut. Interestingly, P.a -infected D. melanogaster flies feeding constantly on 2AA retain more bacteria in their intestine 1 or 2 weeks post infection ( Fig. 4a ). Despite having more bacteria over time, 2AA-treated flies survived infection at least as long as untreated infected flies ( Fig. 4b ). Thus bacteria that produce 2AA may not only attract and contaminate flies, but they might also establish a higher level of colonization in the flies they attract 1 or 2 weeks post infection. 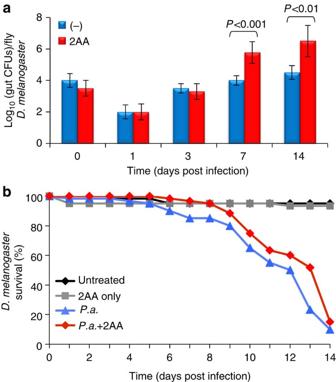Figure 4: Long-term colonization and survival ofP. aeruginosa-infected flies feeding on 2AA. Bacterial load (a) and survival (b) ofD. melanogasterfed withP. aeruginosaand maintained on sucrose media with or without 2AA. Fora,n=6 fly samples (three flies per sample) were assessed per condition and time point; error bars represent s.d. Differences inaare statistically significant at 7 and 14 days (usingt-test),P≤0.01. Forb,n=100 flies per condition. Figure 4: Long-term colonization and survival of P. aeruginosa -infected flies feeding on 2AA. Bacterial load ( a ) and survival ( b ) of D. melanogaster fed with P. aeruginosa and maintained on sucrose media with or without 2AA. For a , n =6 fly samples (three flies per sample) were assessed per condition and time point; error bars represent s.d. Differences in a are statistically significant at 7 and 14 days (using t -test), P ≤0.01. For b , n =100 flies per condition. Full size image Preference for 2AA and foraging in olfactory organ-mutilated flies To find out which olfactory organ facilitates 2AA attraction, we dissected out the fly antennae, the largest olfactory organs, as well as the fly maxillary palps, the olfactory organs attached to the proboscis of D. melanogaster [22] . We found that, irrespective of the presence of 2AA in the fly food, fewer antennaless, maxillary palpless and especially doubly mutilated antennaless-maxillary palpless flies compared with normal wild type (wt) flies enter the traps. Nevertheless, removal of either antennae or maxillary palps from D. melanogaster does not preclude preference for 2AA, but removal of both organs does ( Fig. 5a ). Similarly, removal of antennae from C. capitata , does not inhibit preference for 2AA, but dissection of both the antennae and the maxillary palps completely precludes preference for 2AA ( Fig. 5b ). Despite being less capable to enter flytraps, antennaless D. melanogaster can forage and survive similar to normal flies, while doubly mutilated flies retain a significant, but diminished, ability to navigate towards food ( Fig. 5c ). 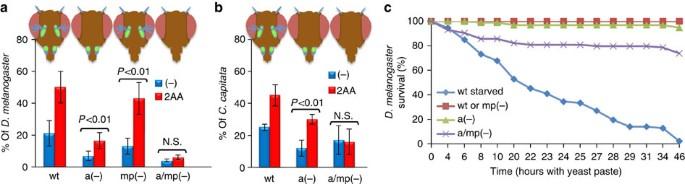Figure 5: Attraction to 2AA and foraging of antennaless and maxillary palpless flies. (a) Attraction of normal (wt), antennaless (a(−)), maxillary palpless (mp(−)) and antennaless–maxillary palpless (a/mp(−))D. melanogasterto yeast paste containing pure 2AA. (b) Attraction of normal (wt), antennaless (a(−)) and antennaless–maxillary palpless (a/mp(−))C. capitatato yeast paste containing pure 2AA. (c) Survival of normal continuously starved (wt starved) as well as normal (wt), antennaless (a(−)), maxillary palpless (mp(−)) and antennaless–maxillary palpless (a/mp(−))D. melanogasterexposed to an open cup containing yeast paste. Inaandb, 100 flies were used per each of then=6 replicates; error bars represent s.d.; organs in green in the inset cartoons indicate existence of antennae and maxillary palps. Differences inaandbare significant (usingt-test) only for normal flies,P<0.01; N.S., not significant. Differences incare statistically significant between starved flies and the rest of the conditions (using log-rank test),P<0.001;n=60 flies per condition. Figure 5: Attraction to 2AA and foraging of antennaless and maxillary palpless flies. ( a ) Attraction of normal (wt), antennaless (a(−)), maxillary palpless (mp(−)) and antennaless–maxillary palpless (a/mp(−)) D. melanogaster to yeast paste containing pure 2AA. ( b ) Attraction of normal (wt), antennaless (a(−)) and antennaless–maxillary palpless (a/mp(−)) C. capitata to yeast paste containing pure 2AA. ( c ) Survival of normal continuously starved (wt starved) as well as normal (wt), antennaless (a(−)), maxillary palpless (mp(−)) and antennaless–maxillary palpless (a/mp(−)) D. melanogaster exposed to an open cup containing yeast paste. In a and b , 100 flies were used per each of the n =6 replicates; error bars represent s.d. ; organs in green in the inset cartoons indicate existence of antennae and maxillary palps. Differences in a and b are significant (using t -test) only for normal flies, P <0.01; N.S., not significant. Differences in c are statistically significant between starved flies and the rest of the conditions (using log-rank test), P <0.001; n =60 flies per condition. Full size image Preference for 2AA in genetically modified flies Similar to olfactory organ-mutilated flies, gene disruption of the common odorant neuron co-receptor Or83b ( orco 1 mutation) [23] reduces the attraction of flies to food and prevents attraction to 2AA ( Fig. 6a ). To identify odorant receptors that facilitate the preference of Drosophila for 2AA, we expressed the odorant receptors Or10a, Or67a, Or49b and Or85a in the antenna and the maxillary palp olfactory neurons using the Or83b-Gal4 driver [24] . We found that Or49b and Or10a increased, while Or85a inhibited attraction to 2AA, which is manifested in a 2:1 ratio in wt control flies ( χ 2 -test, P <0.01; Fig. 6a ). Or10a loss-of-function flies ( Or10a f03694 ) [25] retain their preference for 2AA (18% (±5% s.d.) versus 50% (±10% s.d. )), which indicates that Or10a is not necessary for attraction towards 2AA. Thus many olfactory receptors, including Or49b and Or10a, which are expressed in the antennae [24] , and others expressed in the maxillary palp, might sense 2AA in a redundant manner. 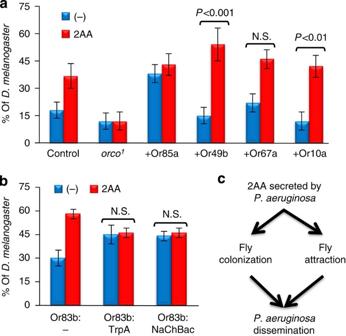Figure 6: Attraction of genetically modified flies to 2AA. (a) Attraction ofD. melanogasteroverexpressing specific odorant receptors in the olfactory organs and oforco1mutant flies severely defected in odour perception to 2AA. (b) Attraction ofD. melanogasteroverexpressing the neuronal activators TrpA or NaChBac in olfactory neurons to 2AA. Thirty to 100 flies were used per each of then=6 replicates; error bars represent s.d.; N.S., not significant. Ratio bias towards 2AA inais higher than 2:1 for Or49b- and Or10a-overexpressing flies (χ2-test,P<0.01). (c) Summary illustration of the two parallel modes of action of 2AA on flies andP. aeruginosa. Figure 6: Attraction of genetically modified flies to 2AA. ( a ) Attraction of D. melanogaster overexpressing specific odorant receptors in the olfactory organs and of orco 1 mutant flies severely defected in odour perception to 2AA. ( b ) Attraction of D. melanogaster overexpressing the neuronal activators TrpA or NaChBac in olfactory neurons to 2AA. Thirty to 100 flies were used per each of the n =6 replicates; error bars represent s.d. ; N.S., not significant. Ratio bias towards 2AA in a is higher than 2:1 for Or49b- and Or10a-overexpressing flies ( χ 2 -test, P <0.01). ( c ) Summary illustration of the two parallel modes of action of 2AA on flies and P. aeruginosa . Full size image Of note, <25% of antennaless or or83b ( orco 1 ) mutant D. melanogaster entered traps compared with >55% of wt flies ( Figs 5a and 6a ). This is to be expected because these defective in odour sensing flies ought to exhibit lower attraction to many of the food odours. On the other hand, ~80% of Or85a overexpressing flies entered traps, but did not show a preference for 2AA. Thus Or85a appears to inhibit the response to 2AA, but not the attraction to other food odours. Interestingly, activating most olfactory neurons in the antennae and maxillary palps using Or83b-Gal4 to express the neuron depolarization proteins TrpA and NaChBac [26] , [27] also inhibits preference for 2AA, but not the overall percentage of flies entering traps ( Fig. 6b ). While massive odorant receptor neuron depolarization is expected to cause defects in olfactory behaviour towards most odorants, in practice we noticed normal attraction to food but loss of attraction towards 2AA. This suggests that constant activation of many olfactory neurons simultaneously may be one way in which 2AA perception can be specifically lost. 2AA is a secondary metabolite of P.a , important in controlling bacterial virulence [18] . Virulence reduction has been correlated with the ability of P.a to chronically colonize humans and animals [18] , [28] . Chronicity is presumably an adaptation that enables the bacteria to live, grow and avoid killing the host for longer periods of time. Accordingly, we found that flies feeding on 2AA- versus no-2AA-containing food are colonized with ~100 times more P.a cells for up to 2 weeks without dying faster from the increased infection. In addition, we showed that a P.a strain that produces 2AA versus an isogenic strain that does not produce 2AA attracts more flies ( D. melanogaster, M. domestica or C. capitata ). Furthermore, we demonstrated that both olfactory organs mediate the fly response to 2AA. Thus, apart from its effect on long-term colonization, 2AA may have evolved to attract and colonize flies facilitating bacterial dissemination ( Fig. 6c ). It is possible that many fly species can sense and respond to 2AA, but those living in an ecosystem that harbours high concentrations of 2AA-producing bacteria are lured to its source. According to the coding of odours by the D. melanogaster odorant receptor repertoire, receptors Or49b, Or10a and Or67a are the only ones shown to respond to many aromatics [24] . Of these three, Or49b and Or10a are more specific in sensing aromatic compounds compared with other types of chemicals [24] . Strikingly, in our experiments these two receptors—but not Or67a—can potentiate 2AA perception. Thus, Or49b and Or10a might increase the sensitivity of olfactory neurons to 2AA. Conversely, Or85a responds to many compounds, including many aromatics to inhibit rather than activate the neurons in which it is expressed [24] . Accordingly, we find that expression of Or85a in olfactory neurons can suppress fly preference for 2AA, suggesting that 2AA or other chemicals in the fly environment might bind to Or85a opposing 2AA-mediated neuron activation. Alternatively, Or85a might activate neurons involved in aversion, similarly to those induced by geosmin [17] . Apart from 2AA, other odorants can also attract flies to their food source. For example, citrus odours increase oviposition, and yeast fermentation odours act as attractants in drosophilids [29] , [30] . Because olfactory neurons in both the fly antennae and maxillary palps can respond to single benzene ring aromatic compounds, such as 2AA [24] , [31] , we propose that odorant receptors in both organs can sense food odours, including 2AA, and thus control attraction to fly food. The pertinent neuronal circuit and concomitant feeding behaviour might be exploitable for the diversion of harmful flies away from human food and into flytraps. Fly stocks Wt Oregon-R and other D. melanogaster strains were reared on cornmeal–yeast–sucrose media at 25 °C. w ; Orco 1 , UAS-TrpA1, UAS-NaChBac and w;Or83b - GAL4 flies were obtained from the Bloomington Stock Center. The latter stock was crossed with w;Δhalo, w;Δhalo;UAS-Or85a, w;Δhalo;UAS-Or49b, w;Δhalo;UAS-Or67b or w;Δhalo;UAS-Or10a (obtained from J. Carlson, Yale University) to obtain odorant receptor-overexpressing flies. Wt M. domestica , obtained as pupae from Oregon Feeder Insects, were kept refrigerated before transferring into empty fly bottles at 25 °C for adult fly eclosion. C. capitata strain A71 was reared in yeast–sucrose–cholesterol media according to Loukeris et al . [32] B. oleae flies were collected from the infested fruits of olive trees in Chania, Greece. P. aeruginosa stocks Wt P.a (PA14 strain) and gene deletion mutants pqsA and pqsBC (PA14 strain derivatives) were obtained from the Laurence Rahme lab (Harvard University) and described in Keserwani et al . [18] P.a has been previously shown to express 2AA at low micromolar to milimolar concentrations depending on the culture media and the microbial strain used [19] . Dual fly trap systems For Drosophila experiments, two adjacent 50-ml Falcon tubes bearing a hole of ~1.2 mm in diameter, in the middle of their thermally cut and inverted conical tips (see Fig. 1a ), were placed in a 1-l glass beaker together with 100 CO 2 -anaesthetized female flies and covered with aluminium foil, secured in place with a rubber band. For M. domestica experiments, two adjacent 180-ml square bottom polypropylene bottles (Genesee Scientific Cat#32-130), covered tightly with a 15 × 15-cm whatman paper funnel with a tip opening of 0.5 cm in diameter (see Fig. 2a ), were placed in a 2-l glass beaker together with 30–50 CO 2 -anaesthetized flies and covered with aluminium foil, secured in place with a rubber band. For C. capitata experiments, two adjacent 240-ml glass bottles, covered tightly with a 15 × 15-cm whatman paper funnel or a plastic funnel with a tip opening of 0.5 cm in diameter (see Fig. 2a ), were placed and sealed in a 27-l plexiglass cage together with 100 CO 2 -anaesthetized flies. For wild-caught Drosophila experiments, two 1-l grass traps, hanging ~1 m apart on an olive grove tree in Heraklion, Greece, were filled with 250 ml of 10% molasses diluted in tap water with or without 2AA (1.5 mM). Dead flies were collected 3 days later from the liquid inside the trap and were counted and morphologically identified at the species level under a stereoscope. Media lures in flytraps For choice experiments in which media contained ‘grown P.a ’, a slice of sterile (control) or P.a -contaminated ~1 cm 3 of LB-solid agar medium was placed inside the cap of a 50-ml fly trap. LB agar media were contaminated with 1 μl of an overnight P.a (PA14 strain) liquid culture or with 1 μl of sterile LB medium (control) and incubated at 37 °C for 24 h prior to their placement in traps. For choice experiments in which media contained ‘added P.a ’, 1 ml of yeast paste was placed inside the cap of a 50-ml Falcon trap or at the bottom of a 180-ml plastic or a 240-ml glass bottle trap. Yeast paste was prepared by mixing 2 g of live yeast (Active Dry Yeast, Genesee Scientific Cat.#62–103) in 6 ml of dH 2 O. On the top of the yeast paste 100 μl of P.a (PA14 strain) culture at OD 600 =5 or 100 μl of sterile LB medium (control) were added. For choice experiments in which media contained ‘2AA(−)’ or ‘wt P.a. ’, 1 ml of yeast paste (2 g of live yeast (Active Dry Yeast, Genesee Scientific Cat.#62–103) in 6 ml of dH 2 O) was placed inside the cap of a 50-ml Falcon trap or at the bottom of an 180-ml plastic or a 240 ml glass bottle trap. On the top of the yeast paste in each trap, we added either 500 μl of pqsA -mutant P.a or 500 μl of pqsBC -mutant P.a LB medium culture at OD 600 =5, grown in the presence of 10 μg ml −1 2-Heptyl-3-hydroxy-4(1H)-quinolone (Sigma-Aldrich Cat.#94398). Under these bacterial culturing conditions the pqsA mutant produces wt levels of 2AA, while the pqsBC strain does not produce any detectable 2AA in a liquid LB medium, as previously determined by liquid chromatography/mass spectroscopy analysis [18] . While 2AA is seemingly the only compound not produced by the pqsA versus the pqsBC mutant, there might be additional differentially produced compounds undetected by our previous liquid chromatography/mass spectroscopy analysis [18] . For choice experiments in which media contained pure 2AA, 1 ml of yeast paste (2 g of live yeast (Active Dry Yeast, Genesee Scientific Cat.#62–103) in 6 ml of dH 2 O) was placed inside the cap of a 50-ml Falcon trap or at the bottom of a 180-ml plastic or a 240-ml glass bottle trap. On the top of the yeast paste of one of the two traps, 0.5 μl of pure 2AA (Sigma-Aldrich Cat.#37804, 98% pure) was added, either directly or upon dilution in 100 ml of dH 2 O. For C. capitata experiments, yeast paste was prepared by diluting 2 g of live yeast in 6 ml of 20% sucrose. Assessment of bacterial load associated with flies Sucrose (4%, 180 μl) was added on each of the three 2.3-cm diameter whatman discs (Fisher #09-820AA) placed inside the cap of three 50-ml D. melanogaster traps or at the bottom of a 240-ml glass bottle C. capitata trap. On the top of each disc, 20 μl of a P.a (PA14 strain) LB medium culture at OD 600 =5 was added. The cultures were first centrifuged at 8,000 g for 2 min and bacterial pellets were either suspended on fresh LB medium (no 2AA) or on the LB medium-supernatant that contained 2AA. Twenty female D. melanogaster (Oregon-R) and 25 female C. capitata (A71) flies were transferred inside their respective traps for 24 h and then transferred onto clean traps containing sterile discs soaked in 4% sucrose. Afterwards, the three D. melanogaster - and the three C. capitata -contaminated discs were removed and soaked in 5 ml of LB medium, 50 μl of which was plated in LB agar for disc contamination assessment. These experiments were performed twice. To assess bacterial load outside the flies, live D. melanogaster and C. capitata flies removed from the traps were washed in 100-μl LB and the eluate was plated on LB agar. To assess bacterial load inside the flies, these same flies were briefly immersed in 95% EtOH, dried on a sterile napkin, ground with a 1.5-ml tube pestle and plated onto LB agar. Bacterial colonies formed on plates were enumerated and assessed morphologically following 20 h of incubation at 37 °C. D. melanogaster samples almost exclusively produced colonies of P.a morphology on LB agar plates. C. capitata produced colonies of various morphologies, ~1/10 of which had the typical P.a morphology on LB agar plates. Enumeration of P.a cells in all cases was verified by plating fly eluates and extracts on centrimide agar plates (Sigma-Aldrich Cat.#22470), which are selective media specific for P.a growth. Fly colonization assay upon feeding on 2AA Triplicates of 20 female Oregon-R flies, 5–7-days-old, were fed for 2 days on an ‘infection mix’ added on an autoclaved cotton ball (Genesee Scientific Cat.#51–101) placed at the bottom of a fly vial (Genesee Scientific Cat.#32–120). Each ‘infection mix’ contained 50 μl of P.a (PA14 strain) culture in LB medium at OD 600nm =2, added in 5 ml of 4% sucrose. The flies were then incubated at 25 °C. Infected flies were transferred into 50-ml Falcon tubes perforated eight times along their length with a heated 0.9-mm needle to enable aeration, while the cup was perforated four times with a heated 1.2-mm needle and covered with a 2.3-cm whatman disc (Fisher #09-820AA). Sucrose solution (4%, 0.2 ml) with or without 2AA (1.5 mM) were added onto the whatman disc and covered with parafilm to provide food to the flies while reducing contamination of the food by the flies. New fly tubes were prepared daily and flies were incubated at 25 °C. To assess bacterial load inside the flies, live flies were briefly immersed in 95% EtOH, dried on a sterile napkin, ground with a 1.5-ml tube pestle and plated onto LB agar. Only live flies were used because dead flies desiccate within hours and bacterial load is gradually eliminated. Statistics Statistical analysis of bacterial load was done using two-tailed Student’s t -test, assuming equal variance. For 2AA versus no-2AA choice experiments, statistical analyses were done using goodness-of-fit χ 2 -test, assessing whether the observed total number of flies in each of the two categories is a random variation of a 1:1 ratio. In addition, we used a χ 2 -test to assess if the observed total number of flies in 2AA versus no-2AA categories for each of the odorant receptor overexpression fly genotypes is a random variation of the 2:1 ratio commonly observed in wt control flies. Where different genotypes were compared these were coded to avoid bias by people performing the assays. For the assessment of differences in fly survival the log-rank test was performed using the MedCalc statistical software. Cleavage of olfactory organs and foraging The antennae and maxillary palps of female D. melanogaster (Oregon-R) and C. capitata were dissected out using forceps under a stereoscope and CO 2 anesthesia. Control non-dissected flies were also anaesthetized under the same conditions. Foraging experiments were performed by placing 24-h starved flies (100 females) in a setup similar to that of flytraps, in which both traps were substituted with an easily accessible 50-ml tube cup containing 3 ml of yeast paste. Wild-caught B. oleae olive fruit sting Ten out of twenty 5-year-old olive trees ( Olea europaea ) growing in pots were sprayed in an open yard with tap water plus 2AA (1.5 mM), while the other ten trees were sprayed with tap water only (control). Each tree was then placed separately in a 1-m 3 plexiglass cage at 25 °C and a 16:8 hour light–dark cycle. On the same day 20 female plus 5 male wild-caught B. oleae were placed inside each cage. All cages contained tap water and 10% sucrose-soaked napkins. On the 6th day, five additional female B. oleae were added in each cage. On the 21st day, all 697 olive fruits were collected from the trees and a total of 1,080 stings were counted. B. oleae were collected from infested olive fruits hanging on olive grove trees in Chania, Greece. The olive fruits were incubated at 25 °C until B. oleae adult eclosion. Three to five day-old-adults were sorted according to sex and distributed into each olive tree cage. How to cite this article: Kapsetaki, S-E. et al . The bacterial metabolite 2-aminoacetophenone promotes association of pathogenic bacteria with flies. Nat. Commun. 5:4401 doi: 10.1038/ncomms5401 (2014).